Quantum networks reveal quantum nonlocality The results of local measurements on some composite quantum systems cannot be reproduced classically. This impossibility, known as quantum nonlocality, represents a milestone in the foundations of quantum theory. Quantum nonlocality is also a valuable resource for information-processing tasks, for example, quantum communication, quantum key distribution, quantum state estimation or randomness extraction. Still, deciding whether a quantum state is nonlocal remains a challenging problem. Here, we introduce a novel approach to this question: we study the nonlocal properties of quantum states when distributed and measured in networks. We show, using our framework, how any one-way entanglement distillable state leads to nonlocal correlations and prove that quantum nonlocality is a non-additive resource, which can be activated. There exist states, local at the single-copy level, that become nonlocal when taking several copies of them. Our results imply that the nonlocality of quantum states strongly depends on the measurement context. Nonlocality is a property of the outcome distributions resulting from local measurements on composite systems. Consider a system shared by N parties, which perform m spacelike separated measurements, with r possible results, on their respective subsystems. Denote by x i =1,..., m the measurement chosen by party i and by a i =1,..., r the corresponding outcome. The obtained joint probability distribution P ( a 1 ,..., a N | x 1 ,..., x N ) is local whenever it can be explained as the result of classically correlated data, represented by λ , following a distribution p ( λ ), that is, Every local distribution (1) satisfies linear constraints known as Bell inequalities. The violation of a Bell inequality is then a signature of nonlocality (distributions not fitting the description (equation (1)) are called nonlocal). Remarkably, local measurements on some quantum states lead to nonlocal correlations [1] . This can be observed in the original Bell test scenario [1] , where the measurements are performed on a single copy of some quantum state ρ . In other words, there exist quantum distributions of outcomes where are the positive operators describing the local measurements by party i , , which cannot be represented by any local model (1). The quantum state ρ is then called nonlocal. Contrary, if the results of all local measurements on ρ can be written as in equation (1), it is local at the single-copy level. A stronger version of nonlocality is possible in a multipartite scenario. Consider the case in which only a subset of the N parties share nonlocal correlations. Although these correlations are nonlocal, they are not genuine N -partite nonlocal. A quantum state is said to be genuine N -partite nonlocal only when there exist measurements on it establishing nonlocal correlations among all the N parties (see Methods). Deciding whether a quantum state is nonlocal not only represents a fundamental question but also has important practical applications. The success of information-processing tasks, as the reduction of communication complexity [2] , no-signalling [3] and device-independent [4] quantum key distribution, device-independent quantum state estimation [5] , [6] or randomness extraction [7] , [8] , crucially relies on the existence of nonlocal correlations. Unfortunately, identifying the nonlocal properties of even the simplest families of entangled quantum state remains an extremely difficult problem [9] , [10] , [11] , [12] . Here, we introduce a new framework to the study of quantum nonlocality. Given an N -partite quantum state ρ , the main idea is to create a network of M ≥ N parties and to distribute among them L copies of ρ , according to a given spatial configuration (see Fig. 1 ). If nonlocal correlations are observed in the network, they must have been provided by the quantum state ρ , which is therefore called nonlocal resource. Within this new scenario, we prove that all one-way entanglement distillable states are nonlocal resources. Then, we construct examples of activation of quantum nonlocality, namely, of quantum states local at the single-copy level, but that become nonlocal in a network scenario, or simply by taking several copies of them. We show that similar activation phenomena occur for genuine multipartite nonlocality. Our results show that quantum networks offer a rich scenario, where the nonlocal properties of quantum states can be better exploited and even activated. 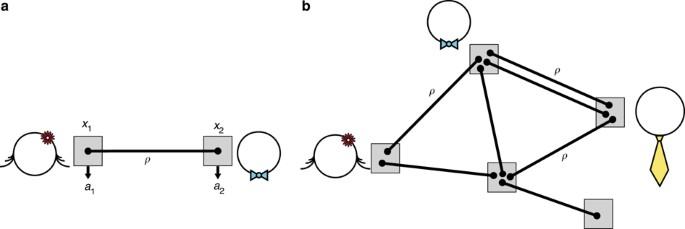Figure 1: Nonlocality in the network scenario. (a) The standard scenario for the study of quantum nonlocality consists ofNparties sharing one copy of anN-party quantum stateρ, to which they applymdifferent measurements ofrpossible results. The measurement choices and corresponding results by the two parties are labelled byx1,...,xN=1,...,manda1,...,aN=1,...,r. By repeating this process, the parties can estimate the joint probability distributionP(a1,...,aN|x1,...,xN) describing the measurement statistics and test its nonlocality. (b) We introduce a new scenario, in which many copies of the quantum stateρare distributed amongMparties according to a network configuration. The parties measure their respective subsystems and check if the obtained multipartite probability distribution is local, that is, if it can be written as in equation (1). As shown in the main text, there are quantum states that are local according to scenarioa, but provide nonlocal correlations in scenariob. Figure 1: Nonlocality in the network scenario. ( a ) The standard scenario for the study of quantum nonlocality consists of N parties sharing one copy of an N -party quantum state ρ , to which they apply m different measurements of r possible results. The measurement choices and corresponding results by the two parties are labelled by x 1 ,..., x N =1,..., m and a 1 ,..., a N =1,..., r . By repeating this process, the parties can estimate the joint probability distribution P ( a 1 ,..., a N | x 1 ,..., x N ) describing the measurement statistics and test its nonlocality. ( b ) We introduce a new scenario, in which many copies of the quantum state ρ are distributed among M parties according to a network configuration. The parties measure their respective subsystems and check if the obtained multipartite probability distribution is local, that is, if it can be written as in equation (1). As shown in the main text, there are quantum states that are local according to scenario a , but provide nonlocal correlations in scenario b . Full size image Framework and tools There exist two main reasons for the network scenario to offer new possibilities in the study of quantum nonlocality. First, it enlarges the standard framework, in which a single-copy of an N -partite state is given to N observers. Joint local measurements become available, which clearly consist of a much more general class of operations than individual local measurements. In fact, joint measurements were already used to reveal some nonlocal properties of quantum states (we will come back to this point in the Discussion). Second, the network scenario allows considering protocols in which a subset of the parties projects the remaining ones into a nonlocal quantum state. Indeed, post-selection is not a valid operation in standard bipartite Bell tests, as it is associated with sending information between the parties. Nevertheless, it is now allowed because it is performed on the results of measurements that are spacelike separated from the measurements actually used in the Bell test (spacelike separation here has the role of time-ordering in the hidden-nonlocality framework [13] , [14] ). These ideas are behind the two main technical observations used next. Consider an N -partite quantum state ρ . Observation 1. If there exist local measurements by k parties such that, for one of the measurement outcomes, the resulting state among the remaining N − k parties is nonlocal, then the initial state ρ is necessarily nonlocal. This fact was first used in ref. 15 to prove that all multipartite entangled pure states are nonlocal. In the Methods, we provide a simple proof of this observation. Observation 2. If, for every bipartition of the parties, there exist local measurements on N −2 parties that, for every outcome, create a maximally entangled state between parties belonging to the different partitions, then the initial state ρ is genuine N -partite nonlocal. This result was proven in ref. 16 and is actually stronger as it also implies that the state ρ strictly contains genuine N -partite nonlocal correlations. Our techniques are fully general and apply to any quantum state. 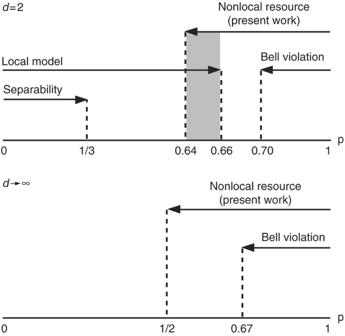Figure 2: Nonlocality of isotropic states. Isotropic states are mixtures of a maximally entangled state and white noise, see equation (3). In the qubit case,d=2, these states violate a Bell inequality forp≳0.705 (ref.28). A local model for any experiment involving von Neumann measurements on a single copy of these states is possible forp≲0.66 (ref.10). This limit also holds if general two-outcome measurements are considered (see Methods (Any two-outcome measurements can be simulated by von Neumann measurements)). In the case of general measurements, the existence of a local model has been proven forp≤5/12 (ref.11). Here, we show, using two-outcome measurements, that two-qubit isotropic states are nonlocal in a network scenario forp≳0.64. In the limit of very large dimension,d→∞, isotropic states violate the Collins–Gisin–Linden–Masar–Popescu (CGLMP) Bell inequality29forp≳0.67. We show that these states are nonlocal resources in our network scenario as soon asp>1/2. However, in what follows, we frequently illustrate their usefulness in networks composed of isotropic states in d × d systems, namely, mixtures of maximally entangled states and white noise, weighted by the noise parameter p : The known nonlocal properties of these states are summarized in Figure 2 . Figure 2: Nonlocality of isotropic states. Isotropic states are mixtures of a maximally entangled state and white noise, see equation (3). In the qubit case, d =2, these states violate a Bell inequality for p ≳ 0.705 (ref. 28 ). A local model for any experiment involving von Neumann measurements on a single copy of these states is possible for p ≲ 0.66 (ref. 10 ). This limit also holds if general two-outcome measurements are considered (see Methods (Any two-outcome measurements can be simulated by von Neumann measurements)). In the case of general measurements, the existence of a local model has been proven for p ≤5/12 (ref. 11 ). Here, we show, using two-outcome measurements, that two-qubit isotropic states are nonlocal in a network scenario for p ≳ 0.64. In the limit of very large dimension, d →∞, isotropic states violate the Collins–Gisin–Linden–Masar–Popescu (CGLMP) Bell inequality [29] for p ≳ 0.67. We show that these states are nonlocal resources in our network scenario as soon as p >1/2. Full size image Any one-way entanglement distillable state is a nonlocal resource We start by showing that any one-way entanglement distillable states form a quantum network that displays nonlocal correlations. The required network consists of three parties in a Λ configuration (see Fig. 3 ): one of the parties, say Alice, shares L copies of ρ with Bob and L additional copies with Charlie. Suppose that ρ is one-way entanglement distillable, using local operations and communication from Alice to each of her partners. In this case, there exists a measurement result by Alice which projects Bob and Charlie into a state that can be made, by increasing L , arbitrarily close to a maximally entangled state. As this state is nonlocal, the network state must be nonlocal by virtue of observation 1. Consequently, nonlocality can be extracted from states which had undetermined nonlocal properties. As an illustration, consider a network made of isotropic states (equation (3)). In the limit of large dimension, nonlocal correlations are observed whenever p >1/2, which is far beyond the known region of Bell violation for the single-copy ρ I (see Fig. 2 ). 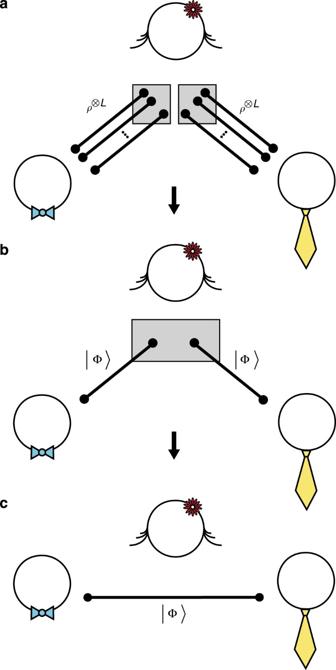Figure 3: Any one-way entanglement distillable state is a nonlocal resource. (a) Consider a network consisting of three distant parties Alice, Bob and Charlie. Alice sharesLcopies of an entangled state with Bob,ρAB, andLcopies of the same state with Charlie,ρAC. (b) Assume this state has non-zero one-way distillable entanglement, using communication from Alice to each partner. Then, there exists a projection on Alice's part ofsuch that the resulting state between Alice and Bob,σAB, tends to a maximally entangled state, in the limit of an infinite number of copies, that is, 〈Φ|σAB|Φ〉→1 whenL→∞. The same projection is applied by Alice to her part of. (c) Alice projects now her subsystems into a maximally entangled state (entanglement swapping). This, in turn, projects Bob and Charlie into a state, which is arbitrarily close to a maximally entangled state. Clearly, all the previous projections by Alice can be seen as a one-shot measurement that, with non-zero probability, leaves Bob and Charlie in a state arbitrarily close to a maximally entangled state. As this state is nonlocal, we conclude that the network state is also nonlocal (observation 1). In the case of isotropic states (equation (3)), this procedure allows the detection of nonlocality forp>1/2 whend→∞. This value is obtained by computing the hashing bound of these states, which is a lower bound on their one-way distillable entanglement30. Figure 3: Any one-way entanglement distillable state is a nonlocal resource. ( a ) Consider a network consisting of three distant parties Alice, Bob and Charlie. Alice shares L copies of an entangled state with Bob, ρ AB , and L copies of the same state with Charlie, ρ AC . ( b ) Assume this state has non-zero one-way distillable entanglement, using communication from Alice to each partner. Then, there exists a projection on Alice's part of such that the resulting state between Alice and Bob, σ AB , tends to a maximally entangled state, in the limit of an infinite number of copies, that is, 〈Φ| σ AB |Φ〉→1 when L →∞. The same projection is applied by Alice to her part of . ( c ) Alice projects now her subsystems into a maximally entangled state (entanglement swapping). This, in turn, projects Bob and Charlie into a state, which is arbitrarily close to a maximally entangled state. Clearly, all the previous projections by Alice can be seen as a one-shot measurement that, with non-zero probability, leaves Bob and Charlie in a state arbitrarily close to a maximally entangled state. As this state is nonlocal, we conclude that the network state is also nonlocal (observation 1). In the case of isotropic states (equation (3)), this procedure allows the detection of nonlocality for p >1/2 when d →∞. This value is obtained by computing the hashing bound of these states, which is a lower bound on their one-way distillable entanglement [30] . Full size image Activation of genuine multipartite nonlocality We now move to the announced examples of activation of quantum nonlocality. Our first example is concerned with genuine multipartite nonlocality and is remarkably simple. Consider a bipartite maximally entangled state |Φ〉, which clearly is not genuine tripartite nonlocal. However, two copies of |Φ〉 disposed in a Λ configuration, as above, compose a network with genuine tripartite nonlocality. The state of the network reads , and is genuine tripartite nonlocal according to observation 2 (actually, it is fully genuine tripartite nonlocal [16] , which makes this activation example even more striking). Such results can be generalized to an arbitrary number of parties: a star-shaped M -party network, in which the central node is connected to the remaining nodes by one copy of a state |Φ〉, is genuine M -partite nonlocal. 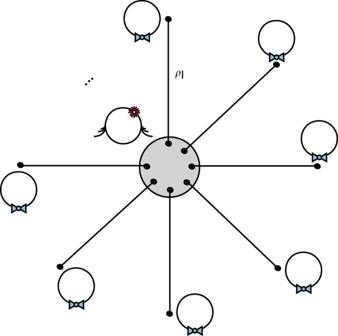Figure 4: Activation of nonlocality. Consider the network scenario in whichN+1 parties share two-qubit isotropic statesρIin a star-like configuration. If the central node, Alice, projects her qubits into the state, the remainingNparties are left with a state that violates a Bell inequality forp>pN=(2/π)21/N(ref.17). It then follows from observation 1 that the network state is nonlocal andρIis a nonlocal resource in this region. ForN≥7, this bound is smaller than the noise corresponding to the best known Bell violation28, that is,p7<0.705. More interestingly, ifN≥21 one haspN<0.66. This is precisely the noise value for which the existence of a local model for von Neumann measurements onρIhas been proven10. As the local model in ref.10can easily be extended to general two-outcome measurements (see Methods) and the previous Bell violation only involved two-outcome measurements, we conclude that the nonlocality ofρIis activated by the network configuration. That is, nonlocal correlations are observed in networks consisting of isotropic states that are local at the single-copy level. Activation of standard quantum nonlocality Moving to standard quantum nonlocality, our example of activation uses isotropic two-qubit states (equation (3)) disposed again in a star-shaped network, as depicted in Figure 4 . In the noise region p ≳ 0.64, there exists a local measurement result in the central node that leaves the remaining subsystems in a nonlocal quantum state [17] . Then, observation 1 guarantees that the corresponding isotropic states are nonlocal resources. But, when p ≲ 0.66, these states are known to be local at the single-copy level for von Neumann measurements [10] (and, consequently, for general dichotomic measurements, see Methods). In the overlap of these regions, quantum nonlocality is activated, that is, local (single-copy) isotropic states form a nonlocal quantum network. The minimal size of the nonlocal network required to enter the single-copy locality region is 21 parties (see caption of Fig. 4 ). Figure 4: Activation of nonlocality. Consider the network scenario in which N +1 parties share two-qubit isotropic states ρ I in a star-like configuration. If the central node, Alice, projects her qubits into the state , the remaining N parties are left with a state that violates a Bell inequality for p > p N =(2/ π )2 1/ N (ref. 17 ). It then follows from observation 1 that the network state is nonlocal and ρ I is a nonlocal resource in this region. For N ≥7, this bound is smaller than the noise corresponding to the best known Bell violation [28] , that is, p 7 <0.705. More interestingly, if N ≥21 one has p N <0.66. This is precisely the noise value for which the existence of a local model for von Neumann measurements on ρ I has been proven [10] . As the local model in ref. 10 can easily be extended to general two-outcome measurements (see Methods) and the previous Bell violation only involved two-outcome measurements, we conclude that the nonlocality of ρ I is activated by the network configuration. That is, nonlocal correlations are observed in networks consisting of isotropic states that are local at the single-copy level. Full size image Activation of quantum nonlocality in the many-copy scenario The examples of activation described previously, network configurations, can be adapted to more standard examples of activation, where the nonlocal properties of a quantum state τ change by simply taking several copies of it, . We call this phenomenon activation of nonlocality in the many-copy scenario. The main idea of our technique is to provide all the parties with classically correlated flags, which allow them to reconstruct the activation network, with a probability that can be made arbitrarily close to one by increasing the number of copies. We illustrate the detailed procedure for the simplest example of activation of genuine multipartite nonlocality; the same construction can be easily applied to the example of activation of standard quantum nonlocality. Consider the tripartite state where and , being |φ〉 some arbitrary state. Clearly this state only has bipartite nonlocal correlations. We show, in what follows, that , for sufficiently large L , is genuine tripartite nonlocal. As said, to do that it is convenient to interpret the qubits in systems A f , B f and C f as flags. Moreover, it is important to recall that two bipartite maximally entangled states in a Λ configuration, , define a genuine tripartite nonlocal state according to observation 2. This means that there exist local measurements by the parties, and , such that the corresponding correlations, described by are genuine multipartite nonlocal, that is, violate a Svetlichny-like Bell inequality [18] , [19] , [20] for the detection of genuine multipartite nonlocality in the no-signalling framework (see discussion in Methods (Definition of genuine multipartite nonlocality)). Given the L copies of σ , the parties apply the following measurement strategies. Alice measures the flag A f of her first copy of σ in the {|0〉,|1〉} basis. Without loss of generality, assume her result is equal to 0. Then, Alice knows she shares a maximally entangled state with Bob in the AB system. She keeps measuring the remaining flags until she gets the outcome 1. In this case, Alice also shares a maximally entangled state with Charlie in the AC systems. That is, she has effectively prepared two singlets in a Λ configuration. Alice now applies the measurement , given in equation (5), to the two particles associated to the two flags in which she first got the results 0 and 1. Bob and Charlie apply a similar strategy: Bob (Charlie) measures the flags B f ( C f ) in the computational basis until he finds result 0 (1). Then he applies the measurement to the corresponding B ( C ) particle. Although presented in a sequential way for clarity reasons, this process defines in fact one-shot local measurements on each party. The obtained correlations among the parties are the same as in equation (5) and, thus, are genuine tripartite nonlocal. Of course, with probability p eq =1/2 L −1 all the flags give the same result. As it becomes clear in the next lines, these instances can be ignored, but we discuss them here for the sake of completeness. Assume that all the flags give 0 (1). Then, the parties can apply, for instance, the measurement strategy on L maximally entangled states between Alice and Bob (Charlie) which optimally approximates P Ψ ( abc | xyz ). The obtained correlations are denoted by , although their explicit form is irrelevant for our considerations. Putting all these possibilities together, the resulting probability distribution among the three parties is equal to This can be made arbitrarily close to the tripartite nonlocal distribution P Ψ ( abc | xyz ), as p eq tends to zero exponentially with the number of copies L . Therefore, there always exists a finite value of L (that might not be large), such that genuine tripartite nonlocal correlations can be obtained from , although σ was not genuine tripartite nonlocal. The example of activation of standard quantum nonlocality can be obtained following a similar procedure. As above, we combine classically correlated flags with the activation result in the network scenario to build an N +1-partite quantum state τ which is local, but such that is nonlocal for large L . The state τ reads where represents the product of a two-qubit isotropic state , shared by parties A and B i , with an arbitrary state for the remaining ones. The states and provide the correlated flags among the parties. Using a similar measurement scheme as above, it is easy to prove that by increasing the number of copies L , can be deterministically transformed into a state arbitrarily close to the nonlocal star-shaped state of Figure 4 . The main ingredient behind activation of quantum resources is the extra capability that each party has of performing local joint operations on particles, uncorrelated among themselves, but, importantly, entangled with some other particles. Clearly, if parties holding several copies of a quantum state only perform individual operations on each particle, they can never obtain a qualitatively different resource from the one already provided by the single-copy state. Several examples have already shown that joint local measurements are useful to enhance the nonlocal properties of some quantum states. Liang and Doherty [21] , for instance, used this strategy to obtain a higher violation of the Clauser–Horne–Shimony–Holt (CHSH) inequality [22] . Recently, Navascués and Vértesi went further: they proved that it is even possible to violate the CHSH inequality with many copies of states that individually are unable to do so [23] . Similar phenomena are observed for the nonlocal content of nonlocal boxes, which are generic (not necessarily physical) devices defined by the probability distributions of their outputs, conditional on the inputs. Still in the context of the CHSH inequality, Forster et al . [24] were the first to prove that it is possible to increase the amount of violation provided by nonlocal boxes, if parties perform local joint operations on several copies of them; and Brunner et al . [25] showed that a similar process can lead to activation of nonlocal properties. The results presented here show that joint measurements allow a drastic extraction of nonlocal resources: there exist quantum states unable to violate any Bell inequality for projective or dichotomic measurements, such that many copies of them allow for the violation of some of these inequalities. Our techniques also show that a much better use of the nonlocal potential of quantum states is achieved simply by distributing them in networks. This work opens then new perspectives in the study of quantum nonlocality. For instance, it would be interesting to analyse if, for any entangled state, there exists a network displaying nonlocal correlations. In fact, despite considerable efforts after Bell's seminal work, we are still far from understanding the exact relation between entanglement and nonlocality [26] , [27] . Our results show that this relation is much subtler than initially expected, the nonlocal character of a quantum state strongly depends on its measurement context, namely, on the network configuration. Definition of genuine multipartite nonlocality In this section, we provide a formal definition of genuine multipartite nonlocality, a stronger version of nonlocality that can be defined in the multipartite scenario [16] , [18] , [19] , [20] . Consider, for instance, a situation in which the correlations observed among N parties can be written as That is, the distribution can be simulated by a hybrid local/nonlocal model, in which nonlocal correlations are given to the first k parties and to the N − k remaining ones, but these two groups are correlated only through the classical random variable λ . Despite the fact that hybrid distributions (equation (9)) can be nonlocal, in the sense of violating equation (1), they are not genuinely multipartite nonlocal, that is, the nonlocal correlations are not shared by all the parties in the system. This observation naturally leads to the concept of genuine N -partite nonlocality. A probability distribution is said to be genuine N -partite nonlocal, or contain genuine N -partite correlations, whenever it cannot be reproduced by the combination of any hybrid models (equation (9)), that is, Here, the terms are such that there exists a splitting of the N parties into two groups, which may depend on λ , allowing a decomposition such as that given in equation (9). Consequently, an N -partite quantum state is said to be genuine N -partite nonlocal whenever there exist local measurement by the parties leading to genuine N -partite nonlocal correlations. It is important to mention here that, throughout this work, we always assume the validity of the no-signalling principle. Thus, all the terms must be compatible with such principle. This does not coincide with the original definition of genuine N -partite nonlocality given in refs [18] , [19] , [20] , but has a natural operational meaning, that is, the parties are assumed not to be able to transmit information instantaneously even if they have access to the variable λ . Similar to standard nonlocality, genuine multipartite nonlocality is usually detected by the violation of some linear inequalities, known as Svetlichny inequalities, that are satisfied by any hybrid local/nonlocal distributions [18] , [19] , [20] . Constructing Bell inequality for N -partite systems In this section, we prove observation 1. The goal, then, is to show that if an N -party state ρ is such that there exist local projections by k parties mapping the remaining N − k parties into a nonlocal state, ρ N − k , then the initial state ρ is also nonlocal. The proof is based on the fact that it is always possible to construct a Bell inequality violated by the state ρ from a Bell inequality violated by the post-measurement nonlocal state ρ N − k . For simplicity in the notation, we consider the case in which the local projections are performed by the first k parties. Take any Bell inequality violated by the nonlocal state ρ N − k , where a = a k +1 ... a N represent the outcomes of the measurements x = x k +1 ... x N performed by the parties k +1,..., N , and c a , x and K are the weights and local bound defining the inequality, respectively. As the state ρ N − k is obtained for a particular outcome of local measurements at parties 1,..., k applied to ρ , we can use equation (11) to write a generalized Bell inequality [15] violated by ρ , Generalized Bell inequalities differentiate from standard ones in the sense that they consider distributions conditioned on particular measurement outcomes, that is, they assume post-selection of events. In general, it is not possible to transform a generalized Bell inequality into a standard Bell inequality. However, this turns out to be possible in our case because the local measurements and results corresponding to the post-selection, y ′ and b ′, define events that are spacelike separated from the measurements appearing in the Bell inequality (11), x . The no-signalling condition then guarantees that the event ( b ′, y ′) can be written independently from measurements x Using this, it directly follows from inequality (12) that the N -partite state ρ must violate which is a standard Bell inequality satisfied by all local models (equation (1)). Any two-outcome measurements can be simulated by von Neumann measurements Here, we show that projective measurements are enough to simulate any outcome distribution obtained by dichotomic (that is, two-outcome) general measurements. Consider a dichotomic measurement described by elements M 0 and M 1 , which are positive operators, such that M 0 + M 1 =1. Then, their spectral decompositions can be expressed in the same basis: and , with 0≤ λ i ≤1. Consequently, the results of this general measurement can be simulated by a protocol consisting of the following steps: (i) the von Neumann measurement defined by projectors {| ϕ i 〉〈 ϕ i |} is applied and (ii) depending on the observed outcome, i , the observer outputs 0 with probability λ i and 1 with probability 1− λ i . This simple observation implies that a local model for projective measurements on a quantum state also applies to general dichotomic measurements. This turns out to be particularly relevant for our example of activation of quantum nonlocality. Recall that this example is based on the fact that the star-shaped network made of isotropic states, see Figure 3 , is nonlocal for a noise threshold p >0.64. It is, however, crucial that dichotomic measurements are sufficient to reveal the nonlocality of the network [17] . Although it is unknown whether there exist isotropic states with p >0.64 that are local under general measurements, as the best known model works for p ≤5/12 (ref. 11 ), they are certainly local for two-outcome measurements when p <0.66. This easily follows from the previous result and the existence of a local model for projective measurements if p <0.66 (ref. 10 ; see Fig. 2 ). We then conclude that isotropic states have their nonlocality activated, that is, there exist states local under dichotomic measurements at the single-copy level, but which have their nonlocality revealed by dichotomic measurements in the network scenario. How to cite this article: Cavalcanti, D. et al . Quantum networks reveal quantum nonlocality. Nat. Commun. 2:184 doi: 10.1038/ncomms1193 (2011).